Haematopoietic cells produce BDNF and regulate appetite upon migration to the hypothalamus Brain-derived neurotrophic factor (BDNF) suppresses food intake by acting on neurons in the hypothalamus. Here we show that BDNF-producing haematopoietic cells control appetite and energy balance by migrating to the hypothalamic paraventricular nucleus. These haematopoietic-derived paraventricular nucleus cells produce microglial markers and make direct contacts with neurons in response to feeding status. Mice with congenital BDNF deficiency, specifically in haematopoietic cells, develop hyperphagia, obesity and insulin resistance. These abnormalities are ameliorated by bone marrow transplantation with wild-type bone marrow cells. Furthermore, when injected into the third ventricle, wild-type bone marrow mononuclear cells home to the paraventricular nucleus and reverse the hyperphagia of BDNF-deficient mice. Our results suggest a novel mechanism of feeding control based on the production of BDNF by haematopoietic cells and highlight a potential new therapeutic route for the treatment of obesity. Brain-derived neurotrophic factor (BDNF), a member of the neurotrophin family, is widely expressed in brain, including in key hypothalamic nuclei known to be important for energy balance regulation [1] , and peripheral tissues, including muscle, liver, adipose and haematopoietic cells [2] , [3] , [4] . Apart from its role in neurotrophic action, BDNF is a central regulator of energy homoeostasis. Intracerebroventricular infusion of BDNF in rodents decreases feeding and body weight [5] , [6] . Conversely, mice that miss a copy of the Bdnf gene develop hyperphagia and obesity [7] , [8] . In humans, genetic haploinsufficiency of BDNF [9] , mutations of the gene encoding its receptor TrkB ( NTRK2 ) [10] and genome-wide association studies [11] , [12] collectively implicate BDNF in the regulation of food intake and obesity development. To identify the origin of BDNF production for energy balance regulation, previous studies focused on either whole brain neurons or specific nuclei in the hypothalamus [13] . Given the recent findings that haematopoietic cells home to brain tissues and that haematopoietic cells express abundant BDNF [2] , [3] , [4] , we examined whether BDNF produced by haematopoietic cells that home to brain tissues participates in energy balance and appetite regulation. Fasting induces migration of haematopoietic cells to the PVN Eight-week-old C57BL/6 mice received whole body irradiation (9 Gy) and bone marrow (BM) transplantation (BMT) from green fluorescent protein (GFP)-transgenic C57BL/6 mice [14] . Eight weeks later, we counted the number of GFP-expressing BM-derived cells in different hypothalamic nuclei under different feeding conditions ( Fig. 1a–c ). We found that BM-derived haematopoietic cells homed to the hypothalamus, specifically in the paraventricular nucleus (PVN), a satiety centre for eating and drinking. Interestingly, fasting (16 or 24 h) led to a significantly increased number of GFP+ cells in the PVN ( Fig. 1b ); the number returned to baseline within 4 h of refeeding following a 16 h fast ( Fig. 1c ). The GFP+ cell density did not change significantly in other hypothalamic nuclei examined ( Fig. 1d ). 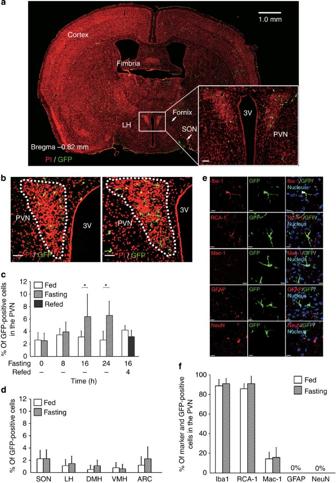Figure 1: Bone marrow-derived cells home to the PVN after fasting. (a) Cerebrum of wild-type mice receiving BMT from GFP-TG mice. Scale bar in lower right panel, 50 μm. LH, lateral hypothalamus; SON, supraoptic nucleus; 3 V, third ventricle. (b) GFP-positive cells in the PVN (delineated by dotted lines) of fed (left) or fasted (16 h, right) mice. Scale bars, 50 μm. (c) Percent of GFP-positive cells in the PVN following fasting (n=3–9). (d) Comparison of GFP-positive cells in other hypothalamic nuclei in fed and fasted mice (n=3–7). DMH, dorsomedial hypothalamus; VMH, ventromedial hypothalamus; ARC, arcuate nucleus. (e) Co-localization of various markers with the GFP-positive cells. Iba1, ionized calcium-binding adaptor molecule 1; RCA-1, ricinus communis agglutinin-1; Mac-1, macrophage antigen complex 1; GFAP, glial fibrillary acidic protein. (f) Percentage of cells positive for both GFP and the indicated markers in the PVN of fed or fasting (16 h) mice (n=4). Scale bars, 10 μm. All data represent the means±s.d. *P<0.05. Figure 1: Bone marrow-derived cells home to the PVN after fasting. ( a ) Cerebrum of wild-type mice receiving BMT from GFP-TG mice. Scale bar in lower right panel, 50 μm. LH, lateral hypothalamus; SON, supraoptic nucleus; 3 V, third ventricle. ( b ) GFP-positive cells in the PVN (delineated by dotted lines) of fed (left) or fasted (16 h, right) mice. Scale bars, 50 μm. ( c ) Percent of GFP-positive cells in the PVN following fasting ( n =3–9). ( d ) Comparison of GFP-positive cells in other hypothalamic nuclei in fed and fasted mice ( n =3–7). DMH, dorsomedial hypothalamus; VMH, ventromedial hypothalamus; ARC, arcuate nucleus. ( e ) Co-localization of various markers with the GFP-positive cells. Iba1, ionized calcium-binding adaptor molecule 1; RCA-1, ricinus communis agglutinin-1; Mac-1, macrophage antigen complex 1; GFAP, glial fibrillary acidic protein. ( f ) Percentage of cells positive for both GFP and the indicated markers in the PVN of fed or fasting (16 h) mice ( n =4). Scale bars, 10 μm. All data represent the means±s.d. * P <0.05. Full size image In these experiments, we created the chimaeric mice by BMT to mice that had received whole body irradiation including the head, a procedure that could have affected the normal vascular function in the brain and enabled an abnormal entry of microglial precursors from blood to the central nervous system (CNS) parenchyma [15] , [16] . To circumvent the possible impact of brain irradiation, we performed a GFP+ BMT experiment in mice that had undergone total body irradiation, in which the head was protected by a lead shield, a strategy that reduced the amount of radiation to the head by 50-fold. In comparison with similar head-protected irradiated fed mice, the number of GFP+ cells in the PVN in 16-h fasted mice was again significantly higher at 220% (fed: 2.5±0.8%; fasted: 5.5±1.9%, mean±s.d., P <0.05 by t -test). Moreover, the 2.5% of GFP+ cells in the PVN of fed mice that had head shielding ( Fig. 1c ) was mildly (~17%) and insignificantly lower than the number in the unshielded group, indicating that the limited effect of head irradiation did not account for the increased presence of GFP+ cells in the PVN of fasted mice. Using similar chimaeric mice, we previously found that electric foot-shock stimulates the influx of cells positive for both GFP and ionized calcium-binding adaptor molecule 1 (Iba1, a CNS microglial marker) into the hippocampus [14] . Therefore, we evaluated the expression of various microglial and nonmicroglial markers in the GFP+ cells ( Fig. 1e ). More than 80% of the GFP+ cells were also positive for Iba1 and ricinus communis agglutinin-1, and fewer than 20% were positive for Mac-1. None of the GFP+ cells were positive for either glial fibrillary acidic protein (an astrocytic marker) or NeuN (a neuronal marker) in fed or fasted mice ( Fig. 1f ). Thus, the GFP+ cells were largely microglia-like. In the previous foot-shock study [14] , some of the GFP+ cells in the hippocampus were positive for major histocompatibility complex-II (MHC-II). We observed that few, if any, GFP+ cells in this study were positive for interleukin (IL)-6, IL-1β, tumour necrosis factor-α or MHC-II ( Supplementary Fig. S1a and S1b ), molecules that are expressed in activated neurotoxic microglia. In addition, we observed that ~40% of the GFP+ cells produced transforming growth factor-β ( Supplementary Fig. S1b ), a microglia-derived factor that supports neuronal survival [17] . Characteristics of haematopoietic cells in the PVN Microglia cells in the spinal cord are known to produce BDNF [18] . Therefore, we tested whether microglial cells in the PVN expressed BDNF. We isolated the microglia-like GFP+ cells from the hypothalamus of both fed and fasted (16 h) mice by laser capture microdissection (LCM; Supplementary Fig. S2 ), and compared their gene expression pattern by microarray analysis and quantified selected transcripts by quantitative real-time–polymerase chain reaction (RT–PCR). We found that the transcripts for a number of genes were upregulated in GFP+ cells in response to fasting. It is noteworthy that some of the upregulated genes had previously been reported to be increased in activated microglia [19] . Specifically, by microarray, compared with control, expression of BDNF mRNA was 220% higher in the fasted mice ( Supplementary Table S1 ). By quantitative RT–PCR, we found that there was a 170% higher BDNF mRNA following fasting. The level of BDNF-mRNA expression was not changed significantly in other hypothalamic nuclei following fasting ( Fig. 2a ). Immunohistochemical analysis revealed that the GFP+ microglial cells also expressed BDNF ( Fig. 2b ). We next determined the percentage of the BDNF+ cells that were microglial in nature (Iba1+) and found that the increase in BDNF+ cells in fasting was accounted for by an increase in the Iba1+ subpopulation of BDNF+ cells ( Fig. 2c and Supplementary Fig. S2c ). As BDNF splice variants are known to be expressed in a highly tissue-specific manner [20] , [21] , we compared the relative expression of different splice variants in the GFP+ cells with that in whole PVN or BM mononuclear cells (BM-MNCs) and found that splice variant type 5 was the major variant produced by the GFP+ cells, and its expression was markedly induced by fasting ( Fig. 2d ). In contrast, whole PVN expressed predominantly variant type 2c, which did not change with fasting. Notably, BM-MNCs expressed the same variant, type 5, that was found in the GFP+ microglial cells. To assess if other noteworthy differences in the gene expression profile of the PVN occurred in fed and fasted mice, we performed microarray analysis of RNA isolated from whole PVN samples obtained by LCM in fed or fasted animals. Interestingly, Cxcl2, a chemokine that regulates haematopoietic mononuclear cell trafficking [22] , was found to be increased >30-fold in the RNA isolated from the PVN of the 16-h fasted mice ( Supplementary Table S2 ), a finding that supports the scenario that fasting-induced Cxcl2 production in the PVN, and the chemokine may then have a role in the trafficking of the GFP+ BM-derived cells [23] , [24] to this region of the hypothalamus. 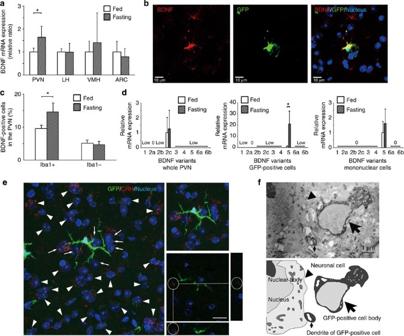Figure 2: Increased hypothalamic expression of BDNF by BMDCs in fasting mice. (a) Comparison of expression of BDNF mRNA in hypothalamic nuclei of fed and fasting mice (n=4–7). (b) Co-localization of BDNF and GFP in the PVN of fasting mice. (c) The percentages of BDNF-positive cells within the Iba1-positive and Iba1-negative cell populations within the PVN (n=6). (d) Comparison of the relative expression of BDNF-mRNA splicing variants in the whole PVN, the GFP-positive cells in the PVN and bone marrow mononuclear cells in fed and fasting mice (n=6–8). Low, low expression. (e) Immunofluorescence laser scanning microscopic analyses of the relative localization of CRH-positive neurons and GFP-positive cells in the PVN of fasting mice. Left panel showed 20-μm thickness accumulated image. The small arrows indicate CRH-positive neurons contacted by the dendrites of single GFP-positive cell in the centre of the panel. Arrowheads showed CRH-positive neurons contacted by GFP-positive cells, whose cell bodies are located outside the plane of this picture. Right lower panel showed 1-μm thickness single slice of right upper 20-μm accumulated image. Narrow pictures were transection ofx- ory-axis broken line of the right lower panel, and circles showed dendrites of a GFP-positive cell. Scale bars, 10 μm. (f) Upper panel: Relation of a GFP-positive cell and a neuron in an electron micrograph from the PVN of fasting mice. Small arrow, dendrite of GFP-positive cell contacted with neuron; big arrow, GFP-positive cell body; arrowhead, margin of a neuron. Lower panel: complementary schematic interpretation of the upper image. All data represent the means ±s.d. Fasting data, fasting for 16 h. *P<0.05. Figure 2: Increased hypothalamic expression of BDNF by BMDCs in fasting mice. ( a ) Comparison of expression of BDNF mRNA in hypothalamic nuclei of fed and fasting mice ( n =4–7). ( b ) Co-localization of BDNF and GFP in the PVN of fasting mice. ( c ) The percentages of BDNF-positive cells within the Iba1-positive and Iba1-negative cell populations within the PVN ( n =6). ( d ) Comparison of the relative expression of BDNF-mRNA splicing variants in the whole PVN, the GFP-positive cells in the PVN and bone marrow mononuclear cells in fed and fasting mice ( n =6–8). Low, low expression. ( e ) Immunofluorescence laser scanning microscopic analyses of the relative localization of CRH-positive neurons and GFP-positive cells in the PVN of fasting mice. Left panel showed 20-μm thickness accumulated image. The small arrows indicate CRH-positive neurons contacted by the dendrites of single GFP-positive cell in the centre of the panel. Arrowheads showed CRH-positive neurons contacted by GFP-positive cells, whose cell bodies are located outside the plane of this picture. Right lower panel showed 1-μm thickness single slice of right upper 20-μm accumulated image. Narrow pictures were transection of x - or y -axis broken line of the right lower panel, and circles showed dendrites of a GFP-positive cell. Scale bars, 10 μm. ( f ) Upper panel: Relation of a GFP-positive cell and a neuron in an electron micrograph from the PVN of fasting mice. Small arrow, dendrite of GFP-positive cell contacted with neuron; big arrow, GFP-positive cell body; arrowhead, margin of a neuron. Lower panel: complementary schematic interpretation of the upper image. All data represent the means ±s.d. Fasting data, fasting for 16 h. * P <0.05. Full size image BDNF-expressing microglia are in contact with PVN neurons Direct injection of BDNF peptides into the mouse PVN suppresses food intake [6] , [25] . To assess whether BDNF-expressing microglia supply the BDNF by making direct contact with neurons in the PVN, we compared the localization of the GFP+ cells and PVN neurons ( Fig. 2e and Supplementary Fig. S3a –c). In fasting but not fed mice, we observed multiple small GFP+ granules with diameters of 0.5–1 micrometres on the surface of corticotrophin-releasing hormone (CRH)-positive neurons ( Supplementary Fig. S3b ). Similar GFP+ structures were also found to be enriched on the surfaces of UCN1+ and AVP+ neurons in fasting mice ( Supplementary Fig. S3a ). Conversely, no significant enrichment of such granules was detected on OXT+, TRH+, UCN2+ or UCN3+ neurons ( Supplementary Fig. S3c, d). Analysis of thick tissue sections by laser scanning microscopy revealed that these GFP+ granules largely represented the tips of dendrites emanating from GFP+ cells ( Fig. 2e ). Importantly, under the laser scanning microscope, we observed that numerous CRH+ neurons (marked by arrowheads in Fig. 2e ) were in contact with GFP+ dendrites of haematopoietic-derived microglia-like cells, whose cell bodies lie outside the plane of the picture. In other words, the effect of BDNF-producing GFP+ cells was amplified by the contacts they made with CRH+ neurons via their multiple GFP+ dendrites. A combination of electron microscopy and confocal microscopy further revealed that these structures were closely associated with the CRH neurons ( Fig. 2e ), findings consistent with BDNF having a key role in the regulation of the hypothalamic–pituitary–adrenal axis [26] . Mice with BM-specific BDNF deletion are hyperphagic and obese Brain microglial cells develop from the primitive macrophages that derive from haematopoietic progenitors in the yolk sac [27] . However, it remains unclear whether the BM progenitors can functionally replace brain BDNF-producing microglial cells in adult animals [28] . To address this issue, we generated mice with congenital deletion of BDNF in BM-derived cells (BM-BDNF−/−), and examined the therapeutic effect on these animals of BDNF+/+-BMT. The BM-BDNF−/− mice were created by crossing B6.129P2-Lyzs tm1(cre)Ifo /J and STOCK Bdnf tm3Jae /J mice ( Fig. 3a ). We confirmed that the microglia of these mice did not express BDNF by comparing immunostaining for BDNF and Iba1 ( Fig. 3b ). We then created GFP-transgenic BM-BDNF−/− mice (GFP-TG/BM-BDNF−/−) and transplanted BM from the latter to the parental BM-BDNF−/− strain. After 8 weeks, we observed many GFP+ cells in the PVN of the BM-BDNF−/− recipients, all of which were negative for BDNF ( Fig. 3c ). Analysis of the GFP+ cells isolated by LCM revealed that they harboured the exon IX deletion of the BDNF gene in their genomic DNA ( Fig. 3d ), and did not express BDNF mRNA ( Fig. 3e ). Compared with control Cre (BM-BDNF+/+) mice, BM-BDNF−/− mice exhibited obesity, and their food and water intake were upregulated from 8 weeks of age until the end of the examination period (56 weeks; Fig. 4a–c ). Twenty-four-week-old male and female BM-BDNF−/− mice exhibited hyperinsulinaemia and glucose intolerance as revealed by intraperitoneal glucose tolerance test ( Fig. 4d ). Furthermore, BM-BDNF−/− mice exhibited decreased O 2 consumption under light and dark conditions ( Fig. 4e ). 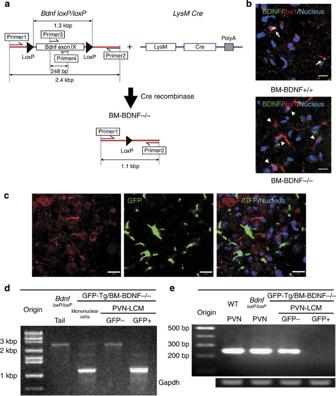Figure 3: Strategy for BM-derived cell (BMDC)-specific BDNF deletion. (a) Schematic of the strategy for the creation of a congenital BDNF deletion specific for BMDCs (BM-BDNF−/−) by the interbreeding of mice of theBdnftm3Jae/J and B6.129P2-Lyzstm1(cre)Ifo/J genotypes. Primers 1 and 2 were designed for the detection of genomic DNA. Primers 3 and 4 were designed for the detection of mRNA. (b) Immunostaining for BDNF and Iba1 in the PVN of BM-BDNF−/− and control LysM-cre mice (BM-BDNF+/+). The arrow indicates co-localization of staining for BDNF and Iba1 in the BM-BDNF+/+ cells, and the arrowhead indicates the lack of such co-localization in the BM-BDNF−/− cells. Scale bars, 10 μm. (c) Analysis of the co-localization of BDNF staining and GFP expression in GFP-TG/BM-BDNF−/− cells. GFP-TG/BM-BDNF−/− mice were generated by interbreeding of GFP-TG and BM-BDNF−/− mice. BDNF did not co-localize with GFP in GFP-TG/BM-BDNF-/- cells. Scale bars, 10 μm. (d) Genomic analysis of BM-BDNF−/−. The 1.3 kb BDNF gene is deleted in mononuclear cells and GFP-positive cells obtained from the PVN of GFP-TG/BM-BDNF−/− mice by LCM. (e) mRNA expression of BDNF. BDNF mRNA was not expressed in GFP-positive cells obtained from the PVN of GFP-TG/BM-BDNF−/− mice by LCM. Figure 3: Strategy for BM-derived cell (BMDC)-specific BDNF deletion. ( a ) Schematic of the strategy for the creation of a congenital BDNF deletion specific for BMDCs (BM-BDNF−/−) by the interbreeding of mice of the Bdnf tm3Jae /J and B6.129P2- Lyzs tm1(cre)Ifo /J genotypes. Primers 1 and 2 were designed for the detection of genomic DNA. Primers 3 and 4 were designed for the detection of mRNA. ( b ) Immunostaining for BDNF and Iba1 in the PVN of BM-BDNF−/− and control LysM-cre mice (BM-BDNF+/+). The arrow indicates co-localization of staining for BDNF and Iba1 in the BM-BDNF+/+ cells, and the arrowhead indicates the lack of such co-localization in the BM-BDNF−/− cells. Scale bars, 10 μm. ( c ) Analysis of the co-localization of BDNF staining and GFP expression in GFP-TG/BM-BDNF−/− cells. GFP-TG/BM-BDNF−/− mice were generated by interbreeding of GFP-TG and BM-BDNF−/− mice. BDNF did not co-localize with GFP in GFP-TG/BM-BDNF-/- cells. Scale bars, 10 μm. ( d ) Genomic analysis of BM-BDNF−/−. The 1.3 kb BDNF gene is deleted in mononuclear cells and GFP-positive cells obtained from the PVN of GFP-TG/BM-BDNF−/− mice by LCM. ( e ) mRNA expression of BDNF. BDNF mRNA was not expressed in GFP-positive cells obtained from the PVN of GFP-TG/BM-BDNF−/− mice by LCM. 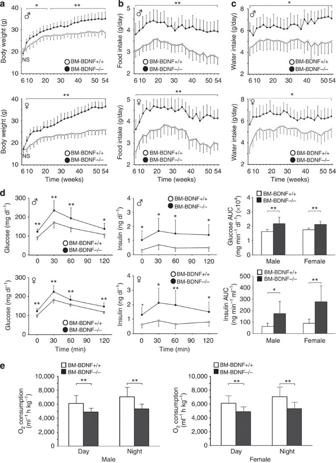Figure 4: BMDC-specific knockout of BDNF. (a–c) Comparison of body weight (a), food intake (b) and water intake (c) in BM-BDNF−/− and control Cre (BM-BDNF+/+) mice (n=10). Upper: male, lower: female. (d) Comparison of glucose and insulin levels, and the corresponding AUC in the intraperitoneal GTT in BM-BDNF−/− and control Cre mice (n=8–11). GTT, glucose tolerance test; AUC, area under the curve. (e) O2consumption of BM-BDNF−/− compared with control Cre mice in light and dark period (n=12). All data represent the means ±s.d. *P<0.05, **P<0.01. Full size image Figure 4: BMDC-specific knockout of BDNF. ( a – c ) Comparison of body weight ( a ), food intake ( b ) and water intake ( c ) in BM-BDNF−/− and control Cre (BM-BDNF+/+) mice ( n =10). Upper: male, lower: female. ( d ) Comparison of glucose and insulin levels, and the corresponding AUC in the intraperitoneal GTT in BM-BDNF−/− and control Cre mice (n=8–11). GTT, glucose tolerance test; AUC, area under the curve. ( e ) O 2 consumption of BM-BDNF−/− compared with control Cre mice in light and dark period ( n =12). All data represent the means ±s.d. * P <0.05, ** P <0.01. Full size image We next took advantage of the different genotypes to examine the distribution of BDNF-mRNA expression in the major hypothalamic nuclei. We quantified in BM-BDNF−/− mice the levels of total and variant 5 BDNF-mRNA expression and compared them with those in Cre BDNF+/+ mice. The haematopoietic-specific BDNF splice variant 5 was below the detection limit in all hypothalamic nuclei in BM-BDNF−/− mouse. In addition, we observed no significant difference in the total BDNF-mRNA expression level in the 16-h fasted vs fed BM-BDNF−/− mice (fasted over fed: 106±10% in the PVN, 92±17% in the LH, 112±11% in the ventromedial hypothalamus (VMH) and 96±9% in the arcuate nucleus (ARC), respectively, n =5). Therefore, the increased BDNF expression in the PVN observed in wild-type fasted mice did not occur in BM-BDNF−/− mice. On the other hand, in comparison with fed Cre mice (BM-BDNF+/+ mice, n =5), the relative levels of total BDNF mRNA in the major hypothalamic nuclei in fed condition in BM-BDNF−/− ( n =5), expressed as % of fed BM-BDNF−/− over fed BM-BDNF+/+, were 84±9% in the PVN, 90±13% in the LH, 97±14% in the VMH and 93±14% in the ARC, respectively. Thus, the levels of expression were significantly reduced only in the PVN ( P <0.05 by t -test), but were not significantly different in the LH, VMH or ARC. In sum, basal BDNF expression in the PVN under basal fed condition was suppressed in BM-BDNF−/− mice, and its fasting-induced upregulation did not happen. Thus, haematopoietic-specific BDNF-mRNA expression has a key role in appetite regulation during a 16-h fast via the PVN. BMT rescues metabolic abnormalities of BDNF deficiency We next performed BMT from GFP-TG/BM-BDNF+/+ or GFP-TG/BM-BDNF−/− donors to BM-BDNF−/− recipients, and then compared fasting-induced PVN homing efficiency ( Supplementary Fig. S4a ) and GFP+ granule formation in the recipient mice ( Supplementary Fig. S4b –e). Interestingly, neither fasting-induced microglial homing nor interaction of the migrated microglia with neurons was affected by BDNF deficiency of the transplanted BM cells. We next examined the therapeutic effect of BMT on BDNF+/+ BM to BM-BDNF−/− mice ( Fig.5a–e ). Food and water intake was significantly decreased in mice that had received BMT from BM-BDNF+/+ mice compared with those that had received BMT from BM-BDNF−/− mice ( Fig. 5b ). At the same time, body weights decreased in both male and female recipients of BDNF+/+ BM as compared with those that had received BDNF−/− BM ( Fig. 5a ). Furthermore, O 2 consumption was increased and glucose intolerance markedly improved in mice that had received BDNF+/+ BM ( Fig. 5d ). 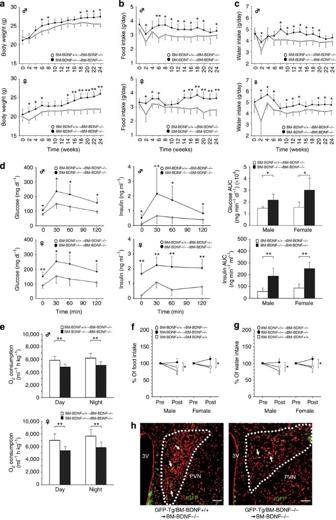Figure 5: BMT and intracerebroventricular BDNF injections in BM-BDNF−/− mice. (a–c) Body weight (a), food intake (b) and water intake (c) in BM-BDNF−/− mice receiving BMT from BM-BDNF+/+ or BM-BDNF−/− mice (n=10). Upper graphs: male, lower: female. (d) Glucose and insulin levels, and the corresponding area under the curve (AUC) 5 months after BMT in the same groups as ina(n=5–6) in GTT. (e) O2consumption 6 months after BMT in the same experimental groups as ina(n=9). Changes in food (f) and water intake (g) following intracerebroventricular injection of mononuclear cells (n=4–6). Data: 7-day average following injection of cells. (h) Microscopic analysis of the injected GFP-positive cells in the PVN. Left panel: BM-MNCs isolated from GFP-Tg/BDNF+/+ mice were injected into the third ventricle (3V) of BM-BDNF−/− mice. Right panel: BM-MNCs isolated from GFP-Tg/BDNF−/− mice were injected. Arrow: GFP-positive cells. Scale bars, 50 μm. All data represent the means±s.d. *P<0.05, **P<0.01,+P=0.06,++P=0.08. Figure 5: BMT and intracerebroventricular BDNF injections in BM-BDNF−/− mice. ( a–c ) Body weight ( a ), food intake ( b ) and water intake ( c ) in BM-BDNF−/− mice receiving BMT from BM-BDNF+/+ or BM-BDNF−/− mice ( n =10). Upper graphs: male, lower: female. ( d ) Glucose and insulin levels, and the corresponding area under the curve (AUC) 5 months after BMT in the same groups as in a ( n =5–6) in GTT. ( e ) O 2 consumption 6 months after BMT in the same experimental groups as in a ( n =9). Changes in food ( f ) and water intake ( g ) following intracerebroventricular injection of mononuclear cells ( n =4–6). Data: 7-day average following injection of cells. ( h ) Microscopic analysis of the injected GFP-positive cells in the PVN. Left panel: BM-MNCs isolated from GFP-Tg/BDNF+/+ mice were injected into the third ventricle (3V) of BM-BDNF−/− mice. Right panel: BM-MNCs isolated from GFP-Tg/BDNF−/− mice were injected. Arrow: GFP-positive cells. Scale bars, 50 μm. All data represent the means±s.d. * P <0.05, ** P <0.01, + P =0.06, ++ P =0.08. Full size image As monocytes and macrophages are present in multiple organs [27] , the deletion of the BDNF gene in response to the Cre activity driven by the LysM promoter might not be restricted to brain microglial cells. We therefore compared the effects of injection of saline or BM-MNCs isolated from GFP-TG/BDNF+/+ or GFP-TG/BM-BDNF−/− mice into the third ventricle of BM-BDNF−/− mice. Within a relatively short period of 8 days of intracerebrovascular injection, during which there was a significant decrease in food ( Fig. 5f ) and water intake ( Fig. 5g ) in the BMT recipients of GFP-TG/BDNF+/+ haematopoietic cells, donor-derived GFP+ BM cells were detectable within the PVN of recipient mice ( Fig. 5h ). Multiple lines of evidence presented in this study indicate that haematopoietic cell-derived BDNF seem to be as important as neuron-derived BDNF in appetite control and obesity in adult animals. In response to a 16-h fast, haematopoietic cells home to the PVN, where they acquire many of the characteristics of microglia and make contact with the local neurons. By producing a haematopoietic-specific variant BDNF, these BM-derived cells regulate food intake via the PVN. It is important to note that the fasting-induced homing of BM-derived cells to the PVN occurs both in total body irradiated mice in the absence or presence of a protective head shield. CNS irradiation per se could cause damage to the vasculature in the brain and allow the abnormal entry of microglial precursors from the circulation to the CNS [15] , [16] . However, we showed that under our experimental conditions, there was only a minor and insignificant increase (~17%) in the number of BM-derived cells that migrated to the PVN in mice without head shield compared with those with head shield. Furthermore, the 16-h fast induced a comparable increase in the number of haematopoietic cells homing to the PVN in head-protected mice vs unprotected irradiated mice. The nature of the signal that stimulates the migration of haematopoietic cells to the PVN requires further investigation. It is intriguing, however, that microarray analysis revealed that the mRNA for Cxcl2, a chemokine produced by endothelial and neural cells, was >30-fold higher in the PVN of fasted compared with fed mice ( Supplementary Table S2 ). Chemokines and cytokines have been implicated in the homing of microglia or BM-derived cells to the nervous system, especially in response to injury or ischaemia in the brain [17] or injury in the spinal cord [29] . Cxcl2 displays potent chemotactic activity towards BM/haematopoietic cell trafficking. Its up-expression in the PVN in these animals could be a trigger for the migration of the BM-derived cells to the PVN during the 16 h fast. This is the initial report on the fasting-induced homing of haematopoietic cells to the PVN, a hypothalamic nucleus, where BDNF produced by these cells can negatively regulate appetite. The potency of BM-derived BDNF on appetite in vivo is evident in BM-BDNF−/− mice, whose failure to respond to fasting by overproducing BDNF in their PVN is manifest in the form of polydipsia, hyperphagia and obesity. Other laboratories have reported that fasting induces an ~50% reduction in BDNF-mRNA level in the VMH [5] , [30] , [31] of mice, a response that would be predicted to lead to an increase in appetite. Importantly, we did not find any change in BDNF expression in the VMH after the 16-h fast. In keeping with this observation, others found that BDNF transcripts do not decrease in the VMH until 48 h into a fast. Appetite control involves a complex network of regulatory nodes that cover different organs of the gastrointestinal system to diverse regions of the brain [32] . The relatively acute recruitment of BDNF-producing haematopoietic cells to the PVN may be a homoeostatic response to the stress of fasting. While it is plausible that the early rise in BDNF in the PVN (via haematopoietic cell homing) may set the stage for a more delayed downregulation of BDNF in the VMH, the exact relationship between the two processes warrants further investigation. We have examined mainly in CRH neurons in this study. However, in the PVN, other neurohormones such as thyrotropin releasing hormone, oxytocin and nesfatin may be involved in the control of feeding and metabolism, and deserve additional investigation in the future. An essential role of haematopoietic expression of BDNF in appetite control is strongly supported by the multiple experiments involving mice that have lost their capability to produce BDNF (and mice with restoration of such capacity) exclusively in BM-derived cells. Recently, BM-derived haematopoietic cells have been found to migrate to the hippocampus following stress induced by foot shocks in mice [14] . Thus, different types of stimuli have been shown to lead to the migration of BM-derived cells to specific regions of the CNS. It is known for decades that haematopoietic mononuclear cells produce BDNF, though the possible function of peripheral cells producing such a potent bioactive molecule has been elusive. Now that we recognize that haematopoietic cells can access specific areas of the CNS in response to various stimuli, we are hopeful that the findings herein energize the discovery of other CNS functions that are potentially regulated by gene products produced by haematopoietic cells. Finally, the revelation of the involvement of the readily accessible haematopoietic cells in appetite control has provided new insight into the pathogenesis of, while it may also accelerate the development of new therapies for, obesity as well as syndromes of appetite dysregulation, such as anorexia nervosa and bulimia. Animals and in vivo studies Mice (C57BL/6 J, C57BL/6-Tg(UBC-GFP)30Scha/J, STOCK Bdnf tm3Jae/J and B6.129P2-Lyzs tm1(cre)Ifo/J , The Jackson Laboratory) were housed individually, maintained on a 12:12-h light–dark schedule at 23 °C, and given ad libitum access to tap water and standard pellets. Animal care was conducted in accordance with the Guide for Use of Experimental Animals (Shiga University of Medical Science). STOCK Bdnf tm3Jae/J and B6.129P2-Lyzs tm1(cre)Ifo/J were culled by the genotyping protocols. LoxP sites were inserted on each side of the single coding exon IX. STOCK Bdnf loxp/loxp were backcrossed to the C57BL/6 J background, and then crossed with mice expressing the Cre recombinase under the direction of the lysozyme M promoter [33] to generate mice on the C57BL/6 J background. To determine Cre-mediated recombination, DNA was extracted from the tail, mononuclear cells, and GFP-negative and positive cells in the PVN by LCM. We designed a PCR primer: Primer 1; 5′-TGTGATTGTGTTTCTGGTGAC-3′ and Primer 2; 5′-TCACTGTTTTCCATGAGTGTCA-3′ ( Fig. 3a ). We extracted mRNA from the PVN of C57BL/6 J mice, the PVN of BDNF loxp/loxp mice, and GFP-negative and GFP-positive cells in the PVN by LCM. After tissue sampling, we synthesized cDNA. We designed a PCR primer: Primer 3; 5′-GCGGCAGATAAAAAGACTGC-3′ and Primer 4; 5′-CTTATGAATCGCCAGCCAAT-3′ ( Fig. 3a ). For BMT, recipient 8-week-old mice were irradiated (9 Gy) and injected with 4 × 10 6 BM cells isolated from donor mice. Eight weeks after BMT, repopulation efficiency by counting the percentage of GFP-positive peripheral white blood cells was determined, and the mice with more than 60% GFP-positive cells were used for the experiments. To protect the brain from radiation, we shielded the head of the mouse by a lead plate during irradiation. Under these conditions, the amount of radiation was dramatically decreased in the region that is shielded with lead, and was less than ~2.2% compared with the site that was not covered by lead plate. We transplanted BM from GFP-transgenic mice to non-GFP mice with radiation with a head shield protection. After 1 month, the transplanted mice were analysed for GFP-positive cells homing to the PVN. At 17:00 hours on the day before mice were killed, access to standard laboratory chow was withdrawn in the fasted group. Mice in the fasted group were separated into individual cages. Brain samples from fed and fasting (16 h) mice were collected at 09:00 hours on the day of the experiment following intraperitoneal administration of 100 mg kg −1 pentobarbital sodium (Nembutal, Abbott Laboratories). Prior to RNA extraction, the brains were frozen in liquid nitrogen and stored at −80 °C. The weight and intake of food and water was determined for the individually caged animals every 2 weeks. Mice were fasted for 5 h, and blood samples were collected for the determination of glucose and insulin. For the glucose tolerance test, mice were injected with glucose (1.5 g kg −1 body weight, intraperitoneally) after fasting for 5 h. We measured the concentration of glucose (Wako Pure Chemical Inds, Osaka, Japan) and serum insulin (Morinaga, Yokohama, Japan). Oxygen consumption was determined by an O 2 /CO 2 metabolism measuring system (Modular Animal Respirometry System, AEI Technologies, Pittsburgh, PA) at 23 °C during the day (08:00–20:00 hours) and night (20:00–08:00 hours). Immunohistochemistry and immunoelectron microscopy Mice were anaesthetized, perfused with 0.01 M phosphate-buffered saline (PBS) to wash out the blood and then perfused with a fixative containing 4% paraformaldehyde, 0.5% glutaraldehyde and 0.2% picric acid in 0.1 M PBS at 4 °C. The brain was immersed for 24 h in postfixative containing 4% paraformaldehyde and 0.2% picric acid in 0.1 M PBS at 4 °C and washed with 0.1 M PBS containing 15% sucrose. Then we cut the brain blocks into 20-μm-thick frozen sections, incubated with primary antibodies listed ( Supplementary Table S3 ), and then incubated with the species-specific secondary antibodies conjugated to FITC, Cy3 (Chemicon) or Texas Red (Vector Laboratories). DAPI (Vector Laboratories), TO-PRO-3 (Molecular Probes) and propidium iodide (PI; Sigma) were used for nuclear staining. TO-PRO-3 was diluted (1:5,000) and the samples were incubated for 10 min on ice. PI staining solution contained PI (50 μg ml −1 ) and RNase (100 μg ml −1 ) (Sigma). The PI-stained samples were incubated for 30 min on 37 °C. Photomicrographs were obtained from 20-μm-thick slices of the specimens observed under a confocal laser scanning microscope (LSM 510, Carl Zeiss, and C1si, Nikon, Japan) or a fluorescence microscope (Biozero, Keyence Japan, Osaka, Japan). The brain samples after the postfixative were embedded in gelatin, and cut into 50-μm-thick sections on a vibratome for immunoelectron microscopy. Immunoreactivity was visualized by reacting with 0.05 M Tris–HCl buffer (pH 7.6) containing 0.01% 3,3′-diaminobenzidine, and 0.0003% H 2 O 2 for 30 min at room temperature. The 3,3′-diaminobenzidine-stained sections were dehydrated, embedded, polymerized and then stained with 2% uranyl acetate before the observation by an electron microscope (H-7100; Hitachi, Japan). Laser capture microdissection and RNA isolation Tissue samples from 12-μm-thick frozen sections for RNA analysis were obtained from each hypothalamic nucleus or 50 captured GFP-positive or -negative cells onto a single CapSure HS LCM Cap (Arcturus Engineering, Mountain View, CA) using the following parameters: spot size=7.5 μm; power=50–80 mW; and pulse duration=50–1,000 μs. Total RNAs were isolated by PicoPure RNA Isolation Kit (Arcturs), and treated with DNase I (Invitrogen). Quantitative RT–PCR We performed quantitative RT–PCR with the LightCycler Fast Start DNA Master SYBR Green I Kit and LightCycler 480 Probe Master (Roche Diagnostics). Emitted fluorescence for each reaction was measured three times during the annealing/extension phase, and the amplification plots were analysed by the use of LIGHT CYCLER 480 System II (Roche Diagnostics). Potential genomic DNA contamination was controlled by the use of some intron-encompassing primers and DNase digestion. The relative value in each sample was calculated by the standard curve obtained from control samples and standardized as the quotient divided by the value simultaneously obtained for glyceraldehyde-3-phosphate dehydrogenase (GAPDH) in the same experiment. The first-strand cDNA was used in subsequent PCR analyses. The following primers were used: BDNF; 5′ upstream primer, 5′-TTGTTTTGTGCCGTTTACCA-3′ and 3′ downstream primer, 5′-GGTAAGAGAGCCAGCCACTG-3′, GAPDH; 5′ upstream primer, 5′-AACGACCCCTTCATTGAC-3′ and 3′ downstream primer, 5′-TCCACGACATACTCAGCAC-3′. The identity of the PCR products was confirmed by size after agarose gel electrophoresis and nucleotide sequence analysis. The signal arising from GAPDH mRNA served as the internal control to evaluate differences among various samples. DNA microarray We captured GFP-positive cells from five different GFP-BMT mice or whole PVN from five wild-type mice both in fed and in fasting (16 h) by LCM. Samples were sent to Bio Matrix Research Laboratory (Japan), where the RNA samples were checked by Agilent 2100 BioAnalyser (Agilent Technologies) and NanoDrop (NanoDrop Technologies). The RNA samples were amplified by two-cycle target labelling, converted to biotinylated cDNA, and hybridized to the Affymetrix Mouse Genome U34A GeneChip array (Santa Clara, CA). We used the Gene Spring Viewer (Agilent Technologies) to analyse the data and calculated the expression ratio ( r =fasting/fed). We showed the expression of microglia-related genes (LCM of GFP-positive cells), and cytokines and inflammation-related genes (LCM of whole PVN) with the result r >2 and r <0.5, although the genes with low expression were excluded from this table ( Supplementary Tables S1 and S2 ), respectively. Hydrolysis probes in RT–PCR for BDNF variants The oligonucleotide primers and hydrolysis probes for real-time reverse transcription–PCR were designed by reference to a previous study [21] ( Supplementary Table S4 ). The amplification was performed with real-time PCR assays using 5′FAM probes (Sigma Genosys) on LIGHT CYCLER 480 System II (Roche Diagnostics). The final reaction volume of 20 μl included 5 μl of cDNA, 0.5 μM of each primer (forward primer and reverse primer), 0.1 μM of 5′FAM probe and 10 μl of LightCycler 480 Probes Master (Roche Diagnostics). Intracerebroventricular injection of mononuclear cells We isolated the mononuclear cell fraction from mouse BM using Ficoll-Paque PLUS (GE Healthcare). After being anaesthesized, the mice head was secured using stereotaxic instruments (SR-6, Scientific Instrument Lab., Tokyo, Japan). Cells were injected into the third ventricle using a 30-G needle attached to a Hamilton syringe according to the coordinates obtained from the textbook by Paxinos and Watson [34] (−0.82 mm from the bregma). The injected volume of the cell suspension was 5 μl and the number of cells per mouse was 1 × 10 6 . Statistical analysis Results are presented as means±s.d. Statistical analysis was performed using SPSS Statistics 19 software. The Student’s t- test was used to compare two independent groups, and the one-way analysis of variance or repeated measure analysis of variance followed by the multiple comparison test was used to compare three or more groups. A statistically significant difference was defined as a P- value<0.05. How to cite this article: Hiroshi U. et al . Haematopoietic cells produce BDNF and regulate appetite on migration to the hypothalamus. Nat. Commun. 4:1526 doi: 10.1038/ncomms2536 (2013).